Empowering a transition-metal-free coupling between alkyne and alkyl iodide with light in water Methods to assemble alkynes are essential for synthesizing fine chemicals, pharmaceuticals and polymeric photo-/electronic materials. Using light as a clean energy form and water as a green solvent has the potential to make synthetic chemistry more environmentally friendly. Here we present a transition-metal-free coupling protocol between aryl alkyne and alkyl iodide enabled by photoenergy in water. Under ultraviolet irradiation and in basic aqueous media, aryl alkynes efficiently couple with a wide range of alkyl iodides including primary, secondary and tertiary ones under mild conditions. A tentative mechanism for the coupling is also proposed. The ongoing pursuit of synthetic efficiency combined with the increasing emphasis on sustainability inspires chemists to explore novel approaches to construct chemical products more efficiently, cleanly, under milder conditions and in an environmentally benign manner [1] , [2] . Although the past several decades have witnessed tremendous successes of transition-metal catalysis in organic chemistry, the difficulty associated with metal residues has led to concerns in, for example, the pharmaceutical and electronic industries. Transition-metal (depleting and precarious) [3] , [4] -free couplings in water (a greener solvent) [5] enabled by photoenergy (a cleaner energy input) [6] provide great opportunities towards more sustainable synthetic chemistry. Alkynes are fundamental structural motifs and are versatile intermediates in chemical transformations [7] , [8] , [9] , [10] , [11] . Research towards the synthesis of alkynes has been pivotal throughout the history of organic chemistry. Methods to synthesize alkyne compounds consist of two types: the first is the direct formation of the triple bond such as the Corey–Fuchs reaction [12] and the Seyferth–Gilbert homologation [13] ; and the second involves modifications on the basis of a pre-existing triple bond [14] , [15] . Diverse metal-catalysed alkyne couplings, including the Glaser–Hay coupling, the Cadiot–Chodkiewicz coupling, the Eglinton coupling, the Castro–Stephens coupling and the Sonogashira coupling, have found wide applications in the synthesis of pharmaceuticals, fine chemicals and polymeric materials [14] . Discovered in 1975, the Sonogashira coupling [16] , owing to its efficiency and robustness, is one of the most reliable reactions to couple terminal alkynes with vinyl/aryl halides or vinyl/aryl pseudohalides. However, the reaction protocol in Sonogashira’s seminal paper is not applicable to the coupling of alkynes with unactivated alkyl halides ( Fig. 1a ). 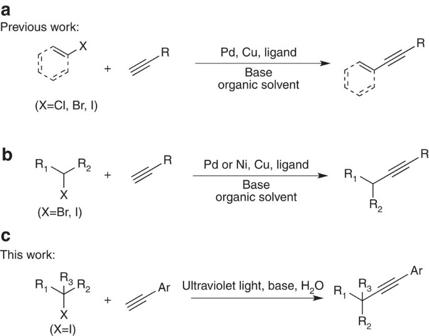Figure 1: Methods for direct alkyne homologation. (a) Classical Sonogashira coupling reaction between an alkyne and an aryl halide. (b) Transition-metal-catalysed coupling of an alkyne with an alkyl halide. (c) Transition-metal-free coupling of an aryl alkyne and an alkyl iodides under ultraviolet in water. Figure 1: Methods for direct alkyne homologation. ( a ) Classical Sonogashira coupling reaction between an alkyne and an aryl halide. ( b ) Transition-metal-catalysed coupling of an alkyne with an alkyl halide. ( c ) Transition-metal-free coupling of an aryl alkyne and an alkyl iodides under ultraviolet in water. Full size image In 2003, Fu et al . [17] pioneered a method of coupling terminal alkynes with unactivated primary bromides and iodides by using catalytic amounts of both palladium and copper salts combined with N-heterocyclic carbene ligands ( Fig. 1b ). Although this method is only suitable for primary bromides and iodides, it inspired chemists to explore other metal/ligand systems to couple more challenging secondary alkyl halides. In ref. 18 , a different protocol was reported, expanding the scope to unactivated secondary bromides and iodides ( Fig. 1b ). Besides palladium, nickel catalysts were also utilized to couple alkynes with unactivated alkyl halides. In 2009, Hu et al . [19] developed a Ni/pincer ligand-based catalyst system to couple terminal alkynes with unactivated primary iodides. By using a catalytic amount of NaI, in situ formation of primary iodides from primary bromides also renders this system applicable to primary bromides ( Fig. 1b ). By further modifying the ligand, Liu et al . [20] reported a protocol capable of coupling alkynes with secondary bromides and iodides under mild conditions ( Fig. 1b ). Along with the Sonogashira-type coupling, other transition-metal-based couplings in the literature such as the Kumada coupling [21] , [22] also allow to synthesize alkyne compounds. However, among all the reports up to now, no known method is available to couple alkynes with unactivated tertiary alkyl halides (whether via classical metal acetylides or modern coupling reactions). Herein, we wish to report the coupling of terminal alkynes with various unactivated alkyl iodides in the absence of any transition metal, assisted by ultraviolet light in water. Most importantly, the method allows the successful coupling of terminal alkynes with tertiary unactivated iodides for the first time ( Fig. 1c ). Designing strategy Before the use of transition metals in synthetic organic chemistry, alkylation of terminal alkynes with alkyl halides via an S N 2 substitution was the traditional technique to construct complex alkyne compounds, in which only primary halides could provide a reasonable yield [23] . Besides the limited substrate scope ( vide supra ), the classical alkylation method also requires a strong base such as n -BuLi or lithium diisopropylamide to pre-generate the metal acetylide [24] ( Fig. 2a,b ). Inspired by Kropp’s seminal work [25] , [26] , [27] , [28] on the heterolytical cleavage of alkyl C–I bond to form carbocations under ultraviolet irradiation in highly polar solvents, we hypothesized that by harmonizing the rate of C–I bond cleavage (related to the light intensity) and the nucleophilicity of the terminal alkyne, the coupling between alkynes and alkyl iodides can be accomplished directly via radical or carbocation intermedates, in the absence of any transiton metals ( Fig. 2c ). 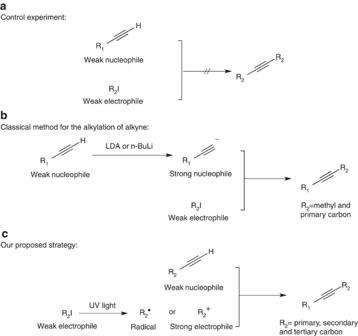Figure 2: Research design. (a) A regular alkyne cannot react with an alkyl halide; (b) the classical coupling of terminal alkyne with the primary halide via metal acetylide; (c) proposed strategy to increase the reactivity of the alkyl halide via radical or carbocation. Figure 2: Research design. ( a ) A regular alkyne cannot react with an alkyl halide; ( b ) the classical coupling of terminal alkyne with the primary halide via metal acetylide; ( c ) proposed strategy to increase the reactivity of the alkyl halide via radical or carbocation. Full size image Optimization of reaction conditions To test our hypothesis, the coupling between 4-methoxyphenylacetylene and cyclohexyl iodide was selected as the model reaction. Extensive investigations were made to optimize the reaction conditions ( Table 1 ). Control experiments ( Table 1 , entries 2 and 3) clearly demonstrated that ultraviolet irradiation is essential for this reaction, as no coupling product was observed without ultraviolet light. Sodium t -butyl oxide as a base was superior to other inorganic and organic bases tested ( Table 1 , entries 5–8 and 12). Addition of inorganic salts ( Table 1 , entry 9) decreased the yield dramatically. Decreasing the amount of cyclohexyl iodide also reduced the yield ( Table 1 , entry 10). Different polar solvents were examined and water was found to be the most beneficial, possibly because of the hydrophobic effect [29] ( Table 1 , entries 4, 11, 15–18, and 25). It is generally accepted that concentration is a key factor in a photoreaction. In our case, either too concentrated or too dilute decreased the product yield, albeit only an emulsion rather than a solution is involved in this reaction system ( Table 1 , entries 19–20). Further confirming that this reaction is transition-metal-free [30] , [31] , [32] , [33] , the addition of 1 equiv CuI actually obstructed the reaction from proceeding ( Table 1 , compare entries 1 and 4 vs 21). By employing different optical filters, ultraviolet light with wavelength <360 nm was found to promote the reaction most efficiently ( Table 1 , entries 22–23). Table 1 Model reaction for the evaluation of different conditions*. Full size table Method applicability With the standard, optimized conditions in hand, we investigated different alkynes and alkyl iodides ( Fig. 3 ). Not unexpectedly, only aryl alkynes underwent coupling effectively at this stage and alkyl alkynes were unreactive under the standard conditions, possibly because aryl alkynes are stronger nucleophiles than alkyl alkynes. However, a triisopropyl-substituted acetylene did generate the desired product successfully, albeit in only 15% yield. Diverse substituents including strong electron-donating groups (for example, -OMe and -NMe 2 ), weak electron-donating groups (for example, -Ph and -alkyl) and electron-withdrawing groups (for example, -F and -CF 3 ) all survived under the reaction conditions, with electron-neutral aryl alkynes giving the best yields (>85%). Besides aryl alkynes, some heteroaromatic alkynes (2-ethynylpyridine and 3-ethynylpyridine) also worked well in this reaction. Aldehyde- and nitro-substituted aryl alkynes were not tolerated under the present conditions, perhaps because of the interference of these functional groups with ultraviolet light. 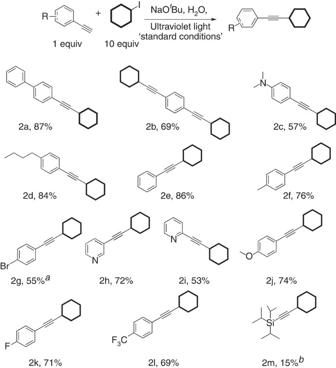Figure 3: Scope of the aryl alkynes. Isolated yield unless otherwise specified;ayield was determined by1H NMR using benzyl alcohol as the internal standard;byield was determined by GC/MS using dodecane as the internal standard. Figure 3: Scope of the aryl alkynes. Isolated yield unless otherwise specified; a yield was determined by 1 H NMR using benzyl alcohol as the internal standard; b yield was determined by GC/MS using dodecane as the internal standard. Full size image As to the scope of electrophiles ( Fig. 4 ), to our surprise, primary (including iodomethane), secondary and even tertiary iodides could all be coupled successfully, among which cyclic secondary alkyl iodides provided the highest yields (52–87%). It should be noted that alkene side products ( ∼ 50% as determined by 1 H NMR) due to elimination was also observed with secondary and tertiary iodides. Many synthetically relevant functional groups such as -Cl, -OTBS (TBS: tert -butyldimethylsilyl) and -NBoc (Boc: tert -butoxycarbonyl), and isolated triple bonds (on the electrophile), were all compatible with the conditions, which provides many opportunities for further structural modifications. 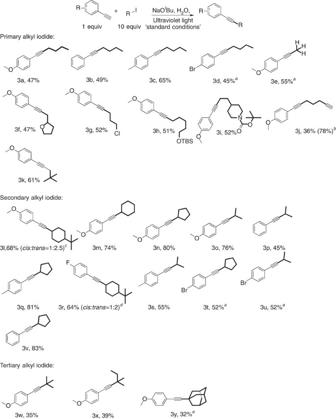Figure 4: Scope of alkyl iodides. Isolated yield unless otherwise specified;ayield was determined by1H NMR analysis through using benzyl alcohol as the internal standard;byield in parentheses was based on recovered starting material;cthecis/transratio was determined through1H NMR analysis of the mixture;dthecis/transratio was determined through1H NMR analysis of the mixture;ethis reaction was conducted in CH3CN. Figure 4: Scope of alkyl iodides. Isolated yield unless otherwise specified; a yield was determined by 1 H NMR analysis through using benzyl alcohol as the internal standard; b yield in parentheses was based on recovered starting material; c the cis/trans ratio was determined through 1 H NMR analysis of the mixture; d the cis/trans ratio was determined through 1 H NMR analysis of the mixture; e this reaction was conducted in CH 3 CN. Full size image During the investigation of the reaction scope, we made a serendipitous discovery of aromatic I–Br exchange. When 4-bromophenylacetylene was employed as the substrate, not only the desired coupling product but also an I–Br exchange compound was detected ( Fig. 5a ). An independent control experiment was executed, in which only bromobenzene and potassium iodide were subjected to ultraviolet irradiation in water ( Fig. 5b ). Iodobenzene, as the iodo–bromo exchange product, was rapidly collected at an unoptimized 40% yield. (See Supplementary Discussion for the details of the I–Br exchange reaction.) This photo-induced aromatic Finkelstein reaction is direct evidence to the existence of the iodide ion, which implied that iodine atom in the alkyl iodide was converted into the iodide ion. Our laboratory is currently conducting further research about this unusual photo-induced transition-metal-free aromatic Finkelstein reaction [34] . 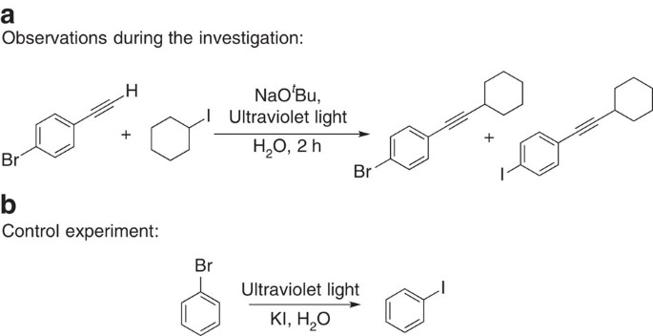Figure 5: Photo-induced aromatic Finkelstein reaction in water. (a) Under standard conditions, the I–Br exchange product was also detected besides the desired coupling product. (b) A control experiment. Figure 5: Photo-induced aromatic Finkelstein reaction in water. ( a ) Under standard conditions, the I–Br exchange product was also detected besides the desired coupling product. ( b ) A control experiment. Full size image To gain more insight regarding the mechanism of this transition-metal-free coupling reaction, further studies were conducted. As shown in Fig. 6 , when cyclopropyl-methyl iodide (a radical clock compound) was subjected to our standard conditions, only the ring-opening coupling compound could be detected, which clearly confirms the existence of a radical intermediate. To further confirm the existence of radical intermediates, (2,2,6,6-tetramethylpiperidin-1-yl)oxy (TEMPO)-trapping investigations were carried out ( Fig. 7 ). The GC/MS (Gas chromatography/mass spectrometry) analysis of the reaction mixture showed the existence of cyclohexyl radical trapped by TEMPO (compound c in Fig. 7 ); however, we failed to detect any radical addition intermediate or its isomers trapped by TEMPO (compound d in Fig. 7 ). Nevertheless, we could not exclude completely the possible involvement of the vinyl radical intermediate. 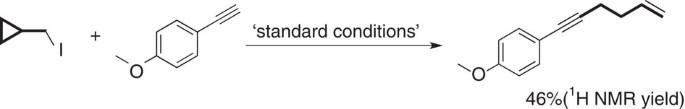Figure 6: Radical clock experiment. Reaction between alkyne substrate and a radical clock compound under standard reaction conditions. Ring-opened product was obatined, implying the existence of radical intermediates. Figure 6: Radical clock experiment. Reaction between alkyne substrate and a radical clock compound under standard reaction conditions. Ring-opened product was obatined, implying the existence of radical intermediates. 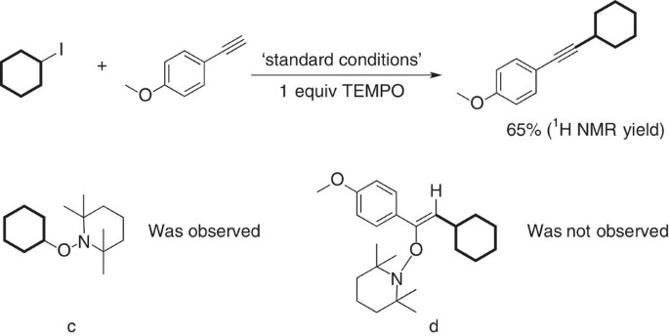Figure 7: TEMPO trapping experiment. Observation of trapped cyclohexyl radical. Full size image Figure 7: TEMPO trapping experiment. Observation of trapped cyclohexyl radical. Full size image On the basis of the results of these studies ( Figs 6 and 7 and Supplementary Discussion ), a tentative mechanism to rationalize the product formation is proposed as follows: the alkyl C–I bond, if homolytically cleaved under ultraviolet light, generates a pair of alkyl and iodine radicals. The alkyl radcial reacts with the alkyne to generate a vinyl radical, which can abstract an iodine atom rapidly either from the alkyl iodide or the free iodine atom in the solution. Finally, a base-promoted E2 reaction of the vinyl iodide produces the desired coupling product ( Fig. 8 ). 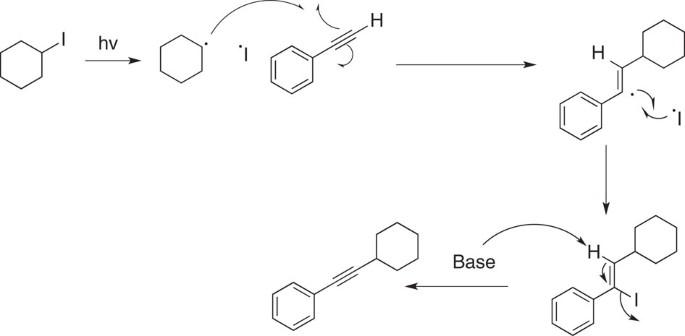Figure 8: Tentative mechanism for the coupling reaction. Radical addition across the triple bond, followed by elimination. Figure 8: Tentative mechanism for the coupling reaction. Radical addition across the triple bond, followed by elimination. Full size image In summary, we have developed a photo-promoted, transition-metal-free protocol to couple aryl alkynes with all types of nonactivated alkyl iodides—including primary, secondary and tertiary—in water for the first time. More importantly, this method allows the direct coupling of terminal alkynes with tertiary iodides. This work not only provides a practical and greener protocol to synthesize alkyne compounds, but also contributes new knowledge to alkyl iodide chemistry. Further studies on the scope, mechanism and synthetic applications of this novel chemistry are under investigation in our laboratory. General protocol of the photo-promoted couplings in water NaO t Bu (80 mg, 0.83 mmol) was added to a 5-ml quartz tube equipped with a rubber septum and a stir bar. Then, 1.5 ml distilled water was added to the tube. After the salt was dissolved and a clear solution was obtained, the solution was degassed and refilled with pre-purified argon three times by using the thaw-frozen technique. Then, 100 μl (0.77 mmol) iodocyclohexane and 10 μl 4-methoxyphenylacetylene (0.077 mmol) were added in succession, which resulted in a two-phase mixture. The rubber septum was quickly replaced by a screw cap and the tube was set in a pre-heated 50 °C water bath. The ultraviolet lamp, located 10 cm away from the tube, was then turned on. Two hours later, the reaction was stopped and EtOAc (3 × 3 ml) was added to extract the organic products. The residue was dried using Na 2 SO 4 and evaporated with a rotavap. Then, the residue was subjected to flush column chromatography on silica gel (Still protocol) by using pure hexane as the eluent to isolate the desired product (12.5 mg, 76% yield, colourless oil). R f value (hexane): 0.12. infrared (cm −1 ): 2,928, 2,853, 2,250, 1,605, 1,508, 1,287, 1,031, 830. 1 H NMR (300 MHz): δ 7.33 (d, J =8.7 Hz, 2H), 6.80 (d, J =8.7 Hz, 2H), 3.80 (s, 3H), 2.59–2.52 (m, 1H), 1.89–1.73 (m, 4H), 1.57–1.33 (m, 3H), 1.33–1.26 (m, 3H); 13 C NMR (75 MHz): 158.9, 132.8, 116.3, 113.7, 92.8, 80.1, 55.2, 32.8, 29.7, 25.9 and 24.9. HRMS-APCI (high resolution mass spectrometry-atmospheric pressure chemical ionization): C 15 H 19 O [M+H] + , calculated: 215.14304, found: 215.14301. For 1 H NMR, 13 C NMR and 19 F NMR (if applicable) spectra of compounds 2a–2m, 3a–3y, see Supplementary Figs 1–65 . For the general information of the analytical methods and the preparation of primary, secondary and tertiary iodides, please see Supplementary Methods . How to cite this article: Liu, W. et al . Empowering a transition metal-free coupling between alkyne and alkyl iodide with light in water. Nat. Commun. 6:6526 doi: 10.1038/ncomms7526 (2015).